Catch-bond mechanism of the bacterial adhesin FimH Ligand–receptor interactions that are reinforced by mechanical stress, so-called catch-bonds, play a major role in cell–cell adhesion. They critically contribute to widespread urinary tract infections by pathogenic Escherichia coli strains. These pathogens attach to host epithelia via the adhesin FimH, a two-domain protein at the tip of type I pili recognizing terminal mannoses on epithelial glycoproteins. Here we establish peptide-complemented FimH as a model system for fimbrial FimH function. We reveal a three-state mechanism of FimH catch-bond formation based on crystal structures of all states, kinetic analysis of ligand interaction and molecular dynamics simulations. In the absence of tensile force, the FimH pilin domain allosterically accelerates spontaneous ligand dissociation from the FimH lectin domain by 100,000-fold, resulting in weak affinity. Separation of the FimH domains under stress abolishes allosteric interplay and increases the affinity of the lectin domain. Cell tracking demonstrates that rapid ligand dissociation from FimH supports motility of piliated E. coli on mannosylated surfaces in the absence of shear force. Cell–cell adhesion often occurs under dynamically varying conditions and mechanical stress. In many cell–cell adhesion systems, the lifetime of adhesin–receptor complexes is increased under tensile mechanical force via ‘catch-bonds’, which permit capture or retention of cells under flow conditions while still allowing for release under reduced mechanical force. Catch-bond interactions are prominent in vascular systems and are formed, for example, by selectins for leukocyte recruitment [1] , [2] , by cadherins controlling tissue integrity [3] , [4] in the epithelial adhesion of cancer cells [5] and by the interactions between T-cell receptors (TCRs) and peptide-bound major histocompatibility complexes (MHC) on antigen-presenting cells [6] , [7] . Catch-bonds also play a major role in bacterial adhesion and infection by uropathogenic Escherichia coli strains, which are responsible for the vast majority of urinary tract infections (UTIs) in humans [8] . A first critical step in the establishment of infection is bacterial adhesion to urothelial cells under flow conditions, which is mediated by 0.1−2 μm long, proteinaceous filaments on the bacterial surface termed type 1 pili [9] , [10] . Type 1 pili are composed of up to 3,000 copies of the subunit FimA building the pilus rod, as well as the subunits FimF, FimG and FimH forming the distal tip fibrillum [11] . The adhesin FimH at the fimbrial tip specifically binds in a catch-bond mode [12] to terminal α- D -linked mannoses of N-linked glycans of the receptor uroplakin 1a on urinary epithelial cells [13] . Owing to its important role in establishing infection, FimH is an attractive target for the development of anti-adhesive drugs for UTI treatment [14] , [15] . FimH is a two-domain protein, composed of an N-terminal, mannoside-binding lectin domain (FimH L ) and a C-terminal pilin domain (FimH P ). FimH P possesses an incomplete immunoglobulin-like fold that is completed by insertion of an N-terminal donor strand of FimG, the subsequent subunit in pilus assembly [11] . The two-domain architecture of FimH is a prerequisite for catch-bond formation because the interactions between FimH L and FimH P determine the conformational state and ligand-binding properties of FimH L (refs 12 , 16 , 17 ). A ‘compressed’ FimH L conformation was observed in the crystal structure of FimH in the context of the type 1 pilus tip fibrillum in the absence of ligands, with an open binding site and interactions to FimH P mediated via three loop segments: the swing (amino acids (aa.) 27–33), linker (aa. 154–160) and insertion loops (aa. 112–118) [17] . In contrast, an ‘extended’ FimH L conformation was observed in crystal structures of the isolated, ligand-bound FimH L domain [18] , [19] , [20] , [21] , [22] , [23] and in the complex between FimH and the pilus assembly chaperone FimC, where FimC prevents the interactions between FimH L and FimH P (ref. 24 ). This extended form of FimH L is characterized by a closed ligand-binding pocket and rearranged swing, linker and insertion loops. Notably, isolated FimH L was reported to show a ligand-binding affinity about two orders of magnitude higher than that of full-length FimH in the tip fibrillum [17] , [25] . Together with mutagenesis experiments disrupting the interdomain interface [26] , these data indicated that ligand-binding is linked to domain separation in FimH, and that mechanical force shifts the ligand-binding affinity towards that of the isolated FimH L . However, fundamental aspects of the mechanism underlying the force-dependent binding of FimH remained unknown: (i) How is domain-associated, full-length FimH interacting with ligands? (ii) Does ligand-binding directly induce domain separation? (iii) How are interdomain interactions linked to the ligand-binding affinity of FimH and the kinetics of ligand-binding and dissociation? To address these questions, we designed a stable, soluble variant of full-length FimH that is equivalent in its structural and functional properties to those of FimH in the assembled fimbrial tip. This variant allowed us to obtain high-resolution structural snapshots of all functional states of FimH and to obtain a complete characterization of ligand-binding kinetics in solution. Together with molecular dynamics simulations, these data reveal a three-state mechanism of FimH catch-bond formation. FimH P accelerates ligand release from FimH L via dynamic allostery by 100,000-fold. In addition, using single-cell tracking experiments, we show that the modulation of ligand affinity by FimH P is not only required for adhesion under mechanical stress, but also for efficient bacterial surface motility in the absence of shear force. Our results provide a first complete structural and kinetic description of a catch-bond system and establish a framework for the analysis of the distinct catch-bond mechanisms in other systems, which also commonly couple interdomain interactions to ligand affinity. Construction of a peptide-complemented FimH Isolated FimH with its non-complemented pilin domain is only marginally stable and shows aggregation tendency under physiological conditions [27] . To establish a stable, isolated FimH molecule with all properties of FimH in the tip fibrillum, we complemented FimH P with the donor-strand peptide of FimG (FimG residues 1−14; termed DsG). The FimH·DsG complex was obtained in good yields and purified after an in vitro reaction, mimicking the first donor-strand exchange (DSE) reaction during pilus assembly in vivo . In this reaction, the FimG donor strand displaces the pilus assembly chaperone FimC from FimH ( Fig. 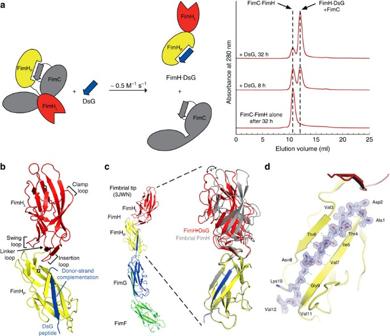Figure 1: FimH·DsG resembles fimbrial tip FimH. (a) Preparation of the FimH·DsG complex by DSE. Left: reaction scheme of the DSE reaction, in which DsG displaces the FimC chaperone from the FimH pilin domain. Right: kinetics of the FimH·DsG complex formation at 37 °C, monitored by analytical gel filtration. DSE was initiated by mixing the FimC·FimH complex (15 μM) with excess DsG peptide (50 μM). Samples were removed after different incubation times, rapidly cooled on ice and immediately subjected to gel filtration. The reaction can be followed by the decrease in the FimC·FimH complex concentration and the simultaneous increase in the concentrations of FimH·DsG and free FimC (FimC and FimH·DsG coelute as a single peak at∼12 ml). The chromatogram at the bottom shows that the FimC·FimH complex is stable against dissociation/aggregation under the chosen conditions. The rate constant of DSE estimated from these data is∼0.5 M−1s−1. (b) Structure of FimHF18·DsG (lectin domain FimHL, red; pilin domain FimHP, yellow; DsG, blue; circle and square indicate N- and C termini, respectively). (c) FimH from the fimbrial tip structure (left, PDB ID: 3JWN (ref.17); FimG, blue; FimF, green) is superposed onto FimHF18·DsG based on their pilin domains (aa. 160–279), in the superposition (right) fimbrial FimH is shown in grey. (d) Close-up on the DsG peptide (stick representation) bound to FimHF18·DsG with 2Fo–Fcelectron density map. Backbone hydrogen bonds of the DsG peptide and β-strands 2 (β2) and 9 (β9) of FimHPare indicated. 1a ): Figure 1: FimH·DsG resembles fimbrial tip FimH. ( a ) Preparation of the FimH·DsG complex by DSE. Left: reaction scheme of the DSE reaction, in which DsG displaces the FimC chaperone from the FimH pilin domain. Right: kinetics of the FimH·DsG complex formation at 37 °C, monitored by analytical gel filtration. DSE was initiated by mixing the FimC·FimH complex (15 μM) with excess DsG peptide (50 μM). Samples were removed after different incubation times, rapidly cooled on ice and immediately subjected to gel filtration. The reaction can be followed by the decrease in the FimC·FimH complex concentration and the simultaneous increase in the concentrations of FimH·DsG and free FimC (FimC and FimH·DsG coelute as a single peak at ∼ 12 ml). The chromatogram at the bottom shows that the FimC·FimH complex is stable against dissociation/aggregation under the chosen conditions. The rate constant of DSE estimated from these data is ∼ 0.5 M −1 s −1 . ( b ) Structure of FimH F18 ·DsG (lectin domain FimH L , red; pilin domain FimH P , yellow; DsG, blue; circle and square indicate N- and C termini, respectively). ( c ) FimH from the fimbrial tip structure (left, PDB ID: 3JWN (ref. 17 ); FimG, blue; FimF, green) is superposed onto FimH F18 ·DsG based on their pilin domains (aa. 160–279), in the superposition (right) fimbrial FimH is shown in grey. ( d ) Close-up on the DsG peptide (stick representation) bound to FimH F18 ·DsG with 2 F o – F c electron density map. Backbone hydrogen bonds of the DsG peptide and β-strands 2 (β2) and 9 (β9) of FimH P are indicated. Full size image The experiments described in the following were performed with FimH from the faecal E. coli strain F18 (FimH F18 ), which is structurally identical to the most prevalent variants in uropathogenic infection [25] , and FimH from the wild-type E. coli strain K12 (FimH K12 ), which differ in three amino acids in FimH L (K12→F18: Val27Ala, Asn70Ser, Ser78Asn; Supplementary Fig. 1a ). The isolated lectin domains (residues 1–159) of both FimH variants (FimH L K12 and FimH L F18 ) were produced by direct expression in the E. coli periplasm and were purified as described [27] . Ligand-free FimH·DsG resembles FimH in the fimbrial tip The crystal structure of the binary complex FimH F18 ·DsG was determined at atomic resolution by molecular replacement ( Table 1 ). FimH F18 ·DsG comprises the jellyroll fold FimH L and the immunoglobulin-like FimH P domain complemented with the FimG donor strand ( Fig. 1b and Supplementary Fig. 1b ). It closely resembles unliganded FimH in the fimbrial tip complex ( Fig. 1c ) [17] , with a root-mean-square deviation of C α positions (C α r.m.s.d.) of 1.1 Å. The individual FimH P and FimH L domains are even more closely resembling unliganded, fimbrial FimH (r.m.s.d. 0.45 and 0.55 Å, respectively) and undergo only a minimal hinge-bending rotation of 4° ( Fig. 1c ). Table 1 Data collection and refinement statistics Full size table The DsG peptide in FimH F18 ·DsG is in identical position as compared with the N-terminal FimG extension in the fimbrial tip structure; it interacts with β-strand 2 and 9 of FimH P ( Fig. 1d ). All contacts in the FimH L –FimH P interdomain region ( Supplementary Fig. 1c,d ) [17] as well as the conformation of the empty ligand-binding pocket observed in FimH in the fimbrial tip are preserved in FimH F18 ·DsG. Thus, FimH F18 ·DsG represents the ligand- free state of fimbrial FimH, with A ssociated FimH L and FimH P ( A free state) and is an elegant minimal system to analyse the crosstalk between ligand-binding and interdomain interactions underlying the formation of catch-bonds by FimH. Persistence of domain association in ligand-bound FimH·DsG To test whether ligand-binding causes domain separation in FimH, we determined the co-crystal structure of the ternary complex of FimH F18 ·DsG with n -heptyl α- D -mannoside (HM), an established model ligand of FimH [20] , as well as crystal structures of the isolated FimH L F18 and FimH L K12 lectin domains in complex with HM ( Table 1 ). FimH F18 ·DsG·HM adopts the same closed conformation of the ligand-binding site as previously observed in other FimH L –ligand complexes ( Fig. 2a,b and Supplementary Fig. 2 ) [28] . The mannopyranose moiety of HM is coordinated by the side chains of Asp54, Gln133, Asn135 and Asp140, and the main chain of Phe1 and Asp47, and the n -heptyl aglycone of HM is sandwiched between Tyr48 and Tyr137. Compared with the A free form, all loops surrounding the binding pocket close down onto the HM ligand. The most substantial conformational difference to A free is observed for the clamp loop (aa. 8–16), whose tip moves almost 6 Å towards HM ( Supplementary Fig. 1e,f ). 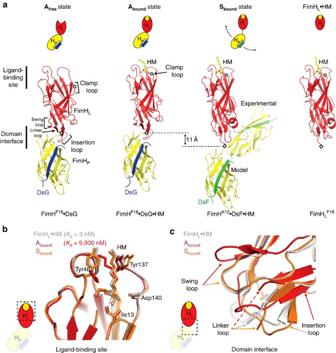Figure 2: Crystallographic analysis of FimH conformational states. (a) FimHF18·DsG in theAfree(left) and in theAboundstates (FimHF18·DsG·HM) in comparison with theSboundstate of FimHK12·DsF·HM and the isolated FimHLF18·HM (right). The FimHL, FimHP, DsF and DsG are coloured in red, yellow, green and blue. The experimentallyin crystallotrapped orientation of FimHPin FimHK12·DsF·HM and a modelled position based on a hinge motion stretching around Gly157 is indicated. A schematic representation for each crystal structure, similar toFig. 1a, is given. The tip of the clamp loop and the C terminus of FimHLare indicated as a circle and diamond, respectively. (b) Comparison of the conformation of the ligand-binding site in theAbound(red) andSbound(orange) states with the isolated lectin domain FimHL(grey) and (c) comparison of the interdomain interface of the lectin domain. Figure 2: Crystallographic analysis of FimH conformational states. ( a ) FimH F18 ·DsG in the A free (left) and in the A bound states (FimH F18 ·DsG·HM) in comparison with the S bound state of FimH K12 ·DsF·HM and the isolated FimH L F18 ·HM (right). The FimH L , FimH P , DsF and DsG are coloured in red, yellow, green and blue. The experimentally in crystallo trapped orientation of FimH P in FimH K12 ·DsF·HM and a modelled position based on a hinge motion stretching around Gly157 is indicated. A schematic representation for each crystal structure, similar to Fig. 1a , is given. The tip of the clamp loop and the C terminus of FimH L are indicated as a circle and diamond, respectively. ( b ) Comparison of the conformation of the ligand-binding site in the A bound (red) and S bound (orange) states with the isolated lectin domain FimH L (grey) and ( c ) comparison of the interdomain interface of the lectin domain. Full size image Besides the closing of the ligand-binding pocket, the overall conformation of ligand-free FimH L in A free and HM-bound FimH F18 ·DsG is closely similar (C α r.m.s.d. 1.1 Å; Fig. 2a,b and Supplementary Fig. 2 ). Unexpectedly, the structural change in the ligand-binding site in FimH F18 ·DsG·HM was not transmitted to the domain interface, where the interdomain contacts and the conformations of the swing, linker and insertion loops remained intact. The lectin domain in the FimH F18 ·DsG·HM complex thus differs drastically from HM-bound isolated FimH L domains with respect to the swing, linker and insertion loop conformations ( Fig. 2c ). On the basis of the persistence of the domain A ssociation in the ligand- bound form, this state of FimH was termed A bound . To test the stability of the A bound state against domain separation and to exclude potential effects of selective crystallization, a molecular dynamics (MD) simulation of the A bound state was conducted using the CHARMM36 force field of the NAMD package ( Supplementary Fig. 3a,b ). The domain association remained intact over 100 ns of simulation time without substantial changes in the domain interface; fluctuations were limited to the clamp loop region close to the ligand-binding site. On in silico removal of the HM ligand after initial equilibration, the A bound state underwent a spontaneous transition to the A free state after ∼ 75 ns of simulation time via an opening of the clamp loop ( Supplementary Fig. 3c,d ), reproducing the experimentally observed dependence of the binding-site conformation on ligand-binding. Thus, the MD simulations indicate that A bound is a stable conformational state of FimH induced by ligand-binding. Trapping of a domain-separated state of full-length FimH The increase in apparent affinity of FimH to its target glycans under tensile mechanical forces [12] , [29] has previously been linked to a separation of the FimH L and FimH P (ref. 17 ). To trap a potential domain-separated state of FimH for structural characterization in the absence of tensile force, we considered FimH variants with weakened interdomain interactions. We had shown previously that FimH P also accepts the donor strand of the non-cognate subunit FimF (DsF). However, FimH P is slightly less stabilized by complementation with DsF than with the natural donor-strand DsG [30] . We hypothesized that such complementation with DsF instead of DsG could also result in a mild destabilization of the interdomain interface in full-length FimH. We then determined the co-crystal structure of FimH K12 ·DsF with HM (FimH K12 ·DsF·HM) at 3.0 Å resolution with four molecules in the asymmetric unit. Three FimH K12 ·DsF·HM molecules closely resembled the A bound state (r.m.s.d. of 0.6 Å to FimH F18 ·DsG·HM) with a preserved interdomain interface. In the fourth molecule, however, the FimH L and FimH P domains were separated and they adopted a drastically different relative orientation with an angle between the domains of ∼ 45° instead of ∼ 150° in the other three molecules ( Fig. 2a ). FimH P is virtually identical in all four FimH molecules in the crystal (r.m.s.d. 0.4 Å). In contrast, the FimH L domain differs significantly between the fourth, domain-separated and the three full-length FimH molecules in the crystal. It shows closest similarity to the isolated FimH L ·HM (r.m.s.d. 0.45 Å); in particular, all interdomain loops adopt identical conformations, which are incompatible with domain association ( Figs 2c and 3 ). Remarkably, in the bent fourth molecule, no interactions between FimH L and FimH P other than the direct covalent linkage are detected, equivalent to a breakdown of the total 500 Å 2 interdomain interface of the A bound state ( Fig. 3 ). This molecule thus represents a third state, the domain- S eparated, ligand- bound state of FimH, S bound . The complete absence of non-covalent interdomain interactions indicates that the S bound state does not possess a defined relative domain orientation in solution, and that the observed, kinked conformation has been selected only by crystal packing. 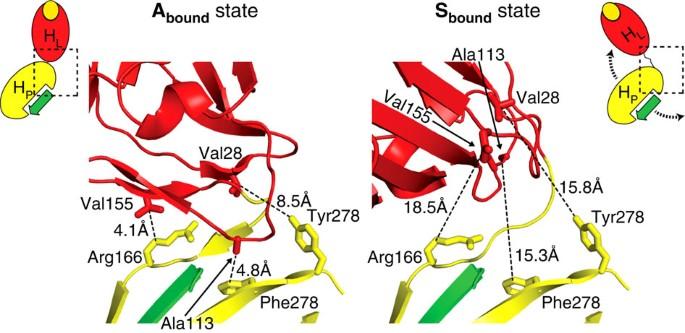Figure 3: The interdomain region in the Sboundstate. Close-up of the interdomain region of FimHK12·DsF·HM in theAboundform (left) and FimHK12·DsF·HM in theSboundstate (right). A cartoon representation for each crystal structure, similar toFig. 1a, is given. Key residues in the interface are shown as sticks. FimHP, FimHLand DsF are coloured in yellow, red and green, respectively. Figure 3: The interdomain region in the S bound state. Close-up of the interdomain region of FimH K12 ·DsF·HM in the A bound form (left) and FimH K12 ·DsF·HM in the S bound state (right). A cartoon representation for each crystal structure, similar to Fig. 1a , is given. Key residues in the interface are shown as sticks. FimH P , FimH L and DsF are coloured in yellow, red and green, respectively. Full size image To analyse the transition trajectory of the A bound to the S bound state, we removed the FimH P domain after equilibration from the A bound state in silico for a 180-ns molecular dynamics simulation ( Supplementary Fig. 3e,f ). In contrast to the transition between the A bound and A free states on ligand removal, a sharp transition to the conformation of FimH L in the S bound state was not observed. The conformation only slowly moved towards S bound ; however, the FimH L loops that had formed in the former interdomain interaction kept fluctuating throughout the simulation, indicating lower cooperativity and potentially a higher activation energy for the A bound → S bound compared with the A bound → A free transition. A comparison of the structural dynamics in the A bound and S bound states clearly reveals differences in the FimH L –FimH P interface region. The root-mean-square fluctuations of atom positions (r.m.s.f.) increase in the swing and insertion loop from a background level of ∼ 0.7 Å in A bound to 1.5 and 2 Å in S bound , respectively. Surprisingly, despite the virtually identical conformations of the entire ligand-binding site depicted by X-ray crystallography ( Fig. 2b ), the clamp loop, which exhibits the most significant conformational changes between the open and closed conformations, exhibits strongly reduced fluctuations in S bound , with r.m.s.f. decreasing by up to 1.5 Å ( Supplementary Fig. 3g,h ). This change in clamp loop dynamics provides a mechanistic link between domain association and ligand-binding in full-length FimH. Domain association alters FimH–ligand-binding kinetics To analyse the ligand-binding properties of FimH·DsG, we exploited the increase in intrinsic tryptophan fluorescence in the FimH·DsG complexes of ∼ 10% on HM binding ( Fig. 4a ). This difference was used to measure the dissociation constant of HM binding by equilibrium titration ( Fig. 4b ) and the rates of HM binding and dissociation by stopped-flow fluorescence kinetics ( Fig. 4c,d ). The FimH·DsG constructs showed uniform binding and dissociation kinetics, consistent with the view that domain-separated states of FimH are not significantly populated in the absence of shear force. The results revealed equilibrium dissociation constants ( K d ) of 3.6 and 9.9 μM for FimH K12 ·DsG and FimH F18 ·DsG, respectively ( Table 2 ). HM binding to FimH·DsG is extremely dynamic and was characterized by fast association rates ( k on ) of 5.0 × 10 6 and 4.9 × 10 6 M −1 s −1 , respectively, and rapid dissociation reactions ( Supplementary Fig. 4 ). The rates of HM dissociation ( k off ) of 22 and 58 s −1 for FimH K12 ·DsG and FimH F18 ·DsG translate into dissociation half-lives of only 32 and 12 ms, respectively. 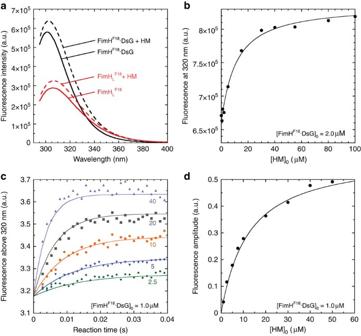Figure 4: Kinetics of HM binding and release by full-length FimH. (a) Fluorescence spectra (excitation at 280 nm) of FimHLF18(2 μM; red lines) and FimHF18·DsG (2 μM; black lines) in the absence (solid lines) or presence of 200 μM HM (dotted lines). (b) Equilibrium titration of FimHF18·DsG (2 μM) with HM, recorded via the fluorescence increase at 320 nm. The total concentration of HM is plotted against the recorded fluorescence signal. Data were fitted (solid line) according to equation (2) (cf.experimental section) and yielded aKdvalue of 9.9±1.5 μM. (c) Stopped-flow fluorescence kinetics of HM binding to FimHF18·DsG (1.0 μM), recorded via the fluorescence change above 320 nm. The HM concentration was varied between 0 and 50 μM. Five representative traces are shown (HM concentrations are given in μM). The fluorescence traces were globally fitted according to a second-order binding and first-order dissociation reaction (solid lines;Table 2). (d) Amplitudes of the reactions monitored inc, plotted against the total HM concentration. Data were fitted (solid line) according to equation (2), yielding aKdvalue of 12±1 μM. Figure 4: Kinetics of HM binding and release by full-length FimH. ( a ) Fluorescence spectra (excitation at 280 nm) of FimH L F18 (2 μM; red lines) and FimH F18 ·DsG (2 μM; black lines) in the absence (solid lines) or presence of 200 μM HM (dotted lines). ( b ) Equilibrium titration of FimH F18 ·DsG (2 μM) with HM, recorded via the fluorescence increase at 320 nm. The total concentration of HM is plotted against the recorded fluorescence signal. Data were fitted (solid line) according to equation (2) ( cf. experimental section) and yielded a K d value of 9.9±1.5 μM. ( c ) Stopped-flow fluorescence kinetics of HM binding to FimH F18 ·DsG (1.0 μM), recorded via the fluorescence change above 320 nm. The HM concentration was varied between 0 and 50 μM. Five representative traces are shown (HM concentrations are given in μM). The fluorescence traces were globally fitted according to a second-order binding and first-order dissociation reaction (solid lines; Table 2 ). ( d ) Amplitudes of the reactions monitored in c , plotted against the total HM concentration. Data were fitted (solid line) according to equation (2), yielding a K d value of 12±1 μM. Full size image Table 2 Kinetics and thermodynamics of HM binding to FimH L or FimH·DsG at pH 7.4 and 25 °C. Full size table In contrast to full-length FimH, isolated FimH L K12 showed no change in tryptophan fluorescence on HM binding. We therefore determined the HM affinity of isolated FimH L indirectly by a competition experiment based on a newly designed fluorescent ligand, the fluorescein-labelled α- D -mannoside GN-FP-4 ( Supplementary Fig. 5a–e and Supplementary Note 1 ). Displacement of GN-FP-4 from FimH L by increasing HM concentrations under equilibrium conditions showed that both FimH L K12 and FimH L F18 bind HM with 3,300-fold higher affinity compared with the respective FimH·DsG complexes ( K d values 1.1 and 3.0 nM, respectively; Fig. 5a and Table 2 ). In an inverse competition experiment ( Supplementary Fig. 5f–j ), in which HM in preformed FimH L ·HM complexes was displaced by GN-FP-4, off-rates of 2.0 × 10 −4 and 3.5 × 10 −4 s −1 were determined for FimH L K12 and FimH L F18 , respectively, corresponding to dissociation half-lives of 58 and 33 min ( Table 2 ). On the basis of these measured off-rates and equilibrium dissociation constants, k on rates of 1.8 × 10 5 and 1.2 × 10 5 M −1 s −1 were calculated for FimH L K12 and FimH L F18 , respectively. The on-rates for the isolated FimH L domains are thus 30-fold lower than those of the corresponding full-length FimH·DsG complexes. 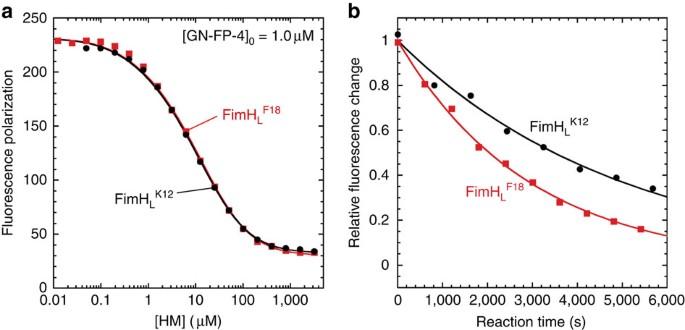Figure 5: HM binding and release by the isolated FimH lectin domain FimHL. Analysis of FimHL·HM interactions based on competition between HM and the synthetic fluorescent GN-FP-4 ligand. (a) HM binding to FimHLanalysed by displacement of GN-FP-4 from FimHLvariants as indicated. An equimolar mixture of FimHLand GN-FP-4 (1 μM each) was incubated with different HM concentrations (10 nM–3.2 mM) for >18 h. GN-FP-4 displacement is monitored by a decrease in fluorescence polarization at 528±20 nm (excitation at 485 nm). Data were fitted (solid lines) according to a mechanism in which two ligands compete for the same binding site, with fixedKdvalues for GN-FP-4 binding (cf.Table 2). (b) Kinetics of HM dissociation from FimHL. A solution with equimolar concentrations of FimHLand HM (3 μM each, guaranteeing >95% occupancy with HM) was mixed with excess GN-FP-4 (10 μM), and the decrease in GN-FP-4 fluorescence at 520 nm as a consequence of HM dissociation and GN-FP-4 binding was recorded (Supplementary Fig. 5f–j). The obtained first-order kinetics are independent of the GN-FP-4 concentration and thus directly monitor HM dissociation. Figure 5: HM binding and release by the isolated FimH lectin domain FimH L . Analysis of FimH L ·HM interactions based on competition between HM and the synthetic fluorescent GN-FP-4 ligand. ( a ) HM binding to FimH L analysed by displacement of GN-FP-4 from FimH L variants as indicated. An equimolar mixture of FimH L and GN-FP-4 (1 μM each) was incubated with different HM concentrations (10 nM–3.2 mM) for >18 h. GN-FP-4 displacement is monitored by a decrease in fluorescence polarization at 528±20 nm (excitation at 485 nm). Data were fitted (solid lines) according to a mechanism in which two ligands compete for the same binding site, with fixed K d values for GN-FP-4 binding ( cf. Table 2 ). ( b ) Kinetics of HM dissociation from FimH L . A solution with equimolar concentrations of FimH L and HM (3 μM each, guaranteeing >95% occupancy with HM) was mixed with excess GN-FP-4 (10 μM), and the decrease in GN-FP-4 fluorescence at 520 nm as a consequence of HM dissociation and GN-FP-4 binding was recorded ( Supplementary Fig. 5f–j ). The obtained first-order kinetics are independent of the GN-FP-4 concentration and thus directly monitor HM dissociation. Full size image Together, these results demonstrate that the 3,300-fold higher affinity of the isolated FimH L compared with full-length FimH results from a more than 100,000-fold lower ligand dissociation rate in isolated FimH L , combined with a ligand-binding rate reduced by only 30-fold ( Table 3 ). The 3,300-fold higher affinity for HM of FimH L relative to FimH·DsG translates into a free energy of 20 kJ mol −1 for the interaction between FimH L and FimH P in full-length FimH. This corresponds very well with the mechanical work required for domain separation, as a displacement of FimH L from FimH P by 11 Å for complete domain separation ( Fig. 2a ) [17] , and a force of 40 pN required to populate the domain-separated state of FimH [31] yields a value of 26.5 kJ mol −1 . Table 3 Comparison of HM binding by variants of FimH L versus FimH·DsG. Full size table Domain association in FimH promotes bacterial motility Uropathogenic E. coli require firm adhesion to the urinary epithelium under flow conditions to escape clearance by urine excretion. On the other hand, bacterial adhesion must be weak enough in the absence of external shear to allow flagellar motility as a prerequisite for the invasion of new tissue areas [32] , [33] . While the role of FimH catch-bond binding for adhesion under flow conditions had clearly been demonstrated [12] , [29] , [34] , the relevance of rapid ligand dissociation under static conditions for flagellar motility remained unclear because of the complex interplay of flagellar swimming and the avidity of multivalent surface interactions by hundreds of E. coli pili. Here we employed single-cell tracking of piliated E. coli cells moving on surfaces coated with mono-mannosylated bovine serum albumin (1M-BSA), an established model system for analysing FimH-based adhesion [12] , [29] , for a classification of cell motility into two states, attached or mobile (for details see Methods and Supplementary Fig. 6 ). To study the influence of FimH interdomain interactions, we compared isogenic E. coli strains producing either wild-type FimH F18 or the FimH F18 -variant Ala188Asp, which is characterized by a destabilized interaction between FimH P and FimH L (ref. 26 ) and serves here to mimic the S bound state in the absence of shear force [35] . The overall fraction of adherent FimH F18 -piliated bacteria on 1M-BSA-coated surfaces was identical to background levels on non-adhesive BSA-coated surfaces at 10–12% of tracked bacteria ( Fig. 6a ). In contrast, FimH F18 –Ala188Asp-piliated bacteria showed an increased fraction of adherent cells of 24% already at the beginning of cell tracking after a 1-min dead time, which further increased during the 5-min observation period to 48% ( Fig. 6a and Supplementary Movies 1 and 2 ). 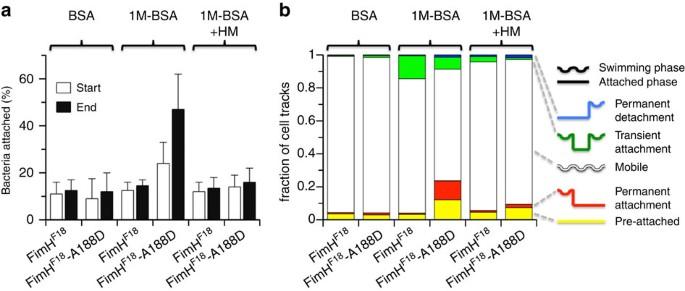Figure 6: Cell-tracking analysis of bacterial motility on mannosylated surfaces. E. colicells piliated with FimHF18or the FimHF18-Ala188Asp variants were tracked under static conditions in the absence of shear force. (a) The fraction of bacteria attached to mannose-coated (1M-BSA) or BSA-coated surface (negative control) at the beginning of the time-lapse movies (white bars) and after 5 min (black bars) are given. Bacterial motility on 1M-BSA was analysed in the absence and presence of HM. The delay between application of bacteria and movie recording was∼1 min. (b) Fraction of tracked cells that were pre-attached (yellow; speed <0.5 μm s−1), permanently attach (red), were mobile (white), transiently attach (green) or permanently detach (blue) during the entire observation time (5 min). Right: schematic depiction of the observed cell behaviour. FimHF18-piliatedE. colishow almost exclusively transient attachment events on 1M-BSA. FimHF18-Ala188Asp-piliatedE. colishow less transient attachment but enhanced permanent attachment to 1M-BSA. Transient and permanent attachment to 1M-BSA is significantly reduced in the presence of HM. For each experiment five to seven independent replicates were analysed. Figure 6: Cell-tracking analysis of bacterial motility on mannosylated surfaces. E. coli cells piliated with FimH F18 or the FimH F18 -Ala188Asp variants were tracked under static conditions in the absence of shear force. ( a ) The fraction of bacteria attached to mannose-coated (1M-BSA) or BSA-coated surface (negative control) at the beginning of the time-lapse movies (white bars) and after 5 min (black bars) are given. Bacterial motility on 1M-BSA was analysed in the absence and presence of HM. The delay between application of bacteria and movie recording was ∼ 1 min. ( b ) Fraction of tracked cells that were pre-attached (yellow; speed <0.5 μm s −1 ), permanently attach (red), were mobile (white), transiently attach (green) or permanently detach (blue) during the entire observation time (5 min). Right: schematic depiction of the observed cell behaviour. FimH F18 -piliated E. coli show almost exclusively transient attachment events on 1M-BSA. FimH F18 -Ala188Asp-piliated E. coli show less transient attachment but enhanced permanent attachment to 1M-BSA. Transient and permanent attachment to 1M-BSA is significantly reduced in the presence of HM. For each experiment five to seven independent replicates were analysed. Full size image Cell tracking permitted quantitative analysis of the transition of individual cells between a mobile and an attached state ( Supplementary Fig. 7 ). On non-adhesive control surfaces coated only with BSA, less than 2% of all FimH F18 - or FimH F18 –Ala188Asp bacteria showed shifts between the two states of motion ( Fig. 6b and Supplementary Fig. 7c ). However, on adhesive 1M-BSA surfaces, 13.9% of all FimH F18 tracks (green in Fig. 6b ) exhibited a single transient attachment event with a mean duration of 6.9 s ( Supplementary Fig. 7d ). For FimH F18 –Ala188Asp-piliated bacteria, only 7.2% of the cells showed attachment/detachment, but with fivefold longer adhesion (35.2 s; Supplementary Fig. 7d ). Remarkably, the fraction of cells that permanently stayed attached after adhesion to 1M-BSA until the end of the observation period was much larger for FimH F18 –Ala188Asp (11.5%) than for FimH F18 (0.6%; red in Fig. 6b ). Those permanently attached cells escape kinetic analysis; thus, the true average attachment time for FimH F18 –Ala188Asp must be considerably larger than 35.2 s. Permanent attachment is also the main cause of the increased fraction of attached cells for FimH F18 –Ala188Asp-piliated bacteria ( Fig. 6a ). Altogether, cell-tracking analysis revealed that enforced domain separation in the FimH F18 –Ala188Asp variant resulted in reduced detachment rates and a larger proportion of permanently attached cells. These results directly demonstrate, at the cellular level, the importance of fast, spontaneous ligand dissociation catalysed by interdomain allostery in FimH–ligand complexes for bacterial motility in the absence of tensile mechanical forces. The characterization of full-length FimH had so far been restricted to the analysis of the adhesive properties of piliated E. coli cells and binding studies with the purified type 1 pilus tip fibrillum. With the FimH·DsG complex, we have now established a model system for quantitative studies of the interaction of FimH with carbohydrate ligands. Soluble FimH·DsG efficiently mimicks FimH in the context of the assembled tip fibrillum, is readily available in milligram quantities and permits the determination of ligand-binding and release kinetics in solution. Using FimH·DsG, we obtained high-resolution snapshots of three functionally relevant states of FimH ( Fig. 7 ). In the absence of ligands, FimH adopts the A free state with associated FimH L and FimH P and an open conformation of the ligand-binding site, which is responsible for the 30-fold faster ligand-binding of full-length FimH as compared with the isolated FimH L domain. Ligand-binding in the absence of shear force induces the A bound state with a closed binding site. In contrast to earlier hypotheses [17] , the transition from A free to A bound is restricted to the ligand-binding site, while all interactions between FimH L and FimH P observed in the A free state remain preserved in A bound . The A free → A bound transition most likely follows an induced fit mechanism, in which the formation of an encounter complex between FimH·DsG and HM is rate-limiting and followed by a fast, unimolecular rearrangement to the A bound state, in agreement with the observation that binding of the model ligand HM remained rate-limiting for the formation of A bound even at the highest HM concentrations used. Stopped-flow-binding kinetics indicate that the lifetime of the proposed encounter complex before A bound formation is below 1 ms ( Fig. 4c ). Under tensile mechanical force applied to the FimH–ligand complex, mimicked here by the destabilized variant FimH·DsF and crystal packing forces, the domain-separated state of FimH, S bound , is formed. In the S bound state, FimH L and FimH P no longer interact specifically and are only connected via the linker segment comprising FimH residues 154–160. In this S bound state, FimH L adopts a conformation closely resembling isolated FimH L with bound ligand. 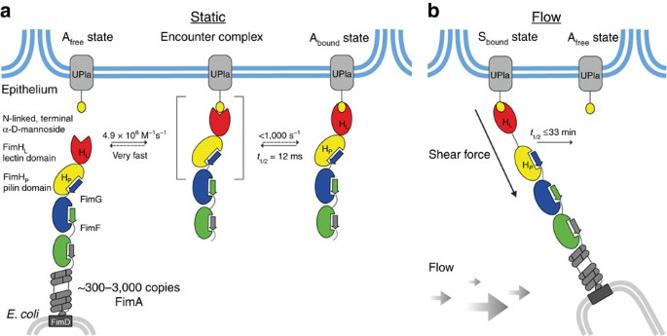Figure 7: Catch-bond mechanism of FimH-mediated cell adhesion. (a) In the absence of tensile mechanical force, formation of the FimH-Uroplakin 1a (UPIa) complex comprises the highly dynamic transition of theAfreeto theAboundstate. The reaction likely proceeds via a transient encounter complex (indicated in square brackets). The reaction of the encounter complex toAboundis not rate-limiting and must have a half-life of less than 1 ms. Dissociation of the receptor from the FimH lectin domain in theAboundstate is promoted via dynamic allostery by the pilin domain that acts as a negative allosteric regulator. The reaction fromAboundto the encounter complex corresponds tokoff. Fast binding and release of UPIa by FimH enables bacterial motility on the bladder epithelium. (b) Shear force increases the population of theSboundstate of FimH, in which the pilin and lectin domains are separated. The dissociation ofSboundunder shear force is slowed down up to 100,000-fold compared withAbound. The indicated rate constants and half-lives correspond to the interaction between FimHF18and the model ligand HM. Rate limiting reactions are indicated by solid arrows, and fast, non-limiting reactions by dashed arrows. Figure 7: Catch-bond mechanism of FimH-mediated cell adhesion. ( a ) In the absence of tensile mechanical force, formation of the FimH-Uroplakin 1a (UPIa) complex comprises the highly dynamic transition of the A free to the A bound state. The reaction likely proceeds via a transient encounter complex (indicated in square brackets). The reaction of the encounter complex to A bound is not rate-limiting and must have a half-life of less than 1 ms. Dissociation of the receptor from the FimH lectin domain in the A bound state is promoted via dynamic allostery by the pilin domain that acts as a negative allosteric regulator. The reaction from A bound to the encounter complex corresponds to k off . Fast binding and release of UPIa by FimH enables bacterial motility on the bladder epithelium. ( b ) Shear force increases the population of the S bound state of FimH, in which the pilin and lectin domains are separated. The dissociation of S bound under shear force is slowed down up to 100,000-fold compared with A bound . The indicated rate constants and half-lives correspond to the interaction between FimH F18 and the model ligand HM. Rate limiting reactions are indicated by solid arrows, and fast, non-limiting reactions by dashed arrows. Full size image Notably, ligand dissociation from FimH·DsG is 100,000-fold faster than that from the isolated FimH L domain. This is striking because the respective crystal structures revealed indistinguishable ligand interactions and binding-site conformations in the FimH·DsG·HM and FimH L ·HM complexes ( Fig. 2b ). MD simulations identified a considerable increase in the conformational dynamics of the FimH L –ligand-enclosing clamp loop in the A bound state as the most likely cause of the dramatic increase in k off in the FimH·DsG·HM complex. The altered dynamics in FimH L in the A bound state are the result of the presence of FimH P , which can be described as a negative allosteric regulator [36] , [37] , [38] . The allosteric communication from the FimH P –FimH L interface to the ligand-binding site reaches over 40 Å, and is mediated via changes in protein dynamics rather than in static structure, in line with a general model of dynamic allostery [39] , [40] . Our data demonstrate that the interdomain interactions in FimH (i) maintain the open conformation of the binding pocket and guarantee rapid ligand-binding and (ii) intramolecularly catalyse ligand dissociation by more than 100,000-fold. Rapid ligand-binding and short lifetimes of the FimH ligand complex allow for rapid dissociation of individual pili from their ligands in the absence of shear force. Our biophysical data demonstrate that this mechanism is conserved between the K12 and the F18 E. coli strains. Different mechanistic models, such as the two-pathway [41] , the deformation [42] and the sliding re-binding model [43] , have been developed to describe catch-bond interactions, often based on powerful single-molecule atomic force measurements. These models included the principle of allosteric control of ligand-binding affinity [26] , [31] , which was clearly fully confirmed in our present study. However, these conceptual models did not reveal the underlying atomic-scale mechanisms in different catch-bond systems. For most catch-bond systems, including the cadherin–catenin binding to actin filaments [3] , [44] , integrin epithelial cell adhesion [45] , [46] and TCR–MHC interactions [6] , [7] , [47] , structural information is, if at all, available only for one state or from computer simulations. One exception is the selectins, which employ catch-bond binding for leukocyte recruitment. Selectins are multidomain cell surface receptors, which consist of a lectin domain for complex carbohydrate binding, linked via an epidermal growth factor (EGF)-like domain to a variable number of short consensus repeat domains and a transmembrane-anchoring helix. Selectins exist in two conformations, a bent and an extended one, which differ in the angle between their lectin and EGF-like domain. Ligand-binding and conformational changes in the ligand-binding site are directly linked via a complex allosteric coupling mechanism to the adoption of the extended conformation [48] , [49] . Tensile mechanical force under flow conditions acts along the axis of the ligand-binding site and the Lec-EGF interface resulting in a stabilization of the extended conformation and thus increased ligand complex lifetimes [2] , [49] . Moreover, in FimH, catch-bond behaviour is mediated by the interplay of a lectin and an anchoring domain that does not interact with the ligand. Ligand-binding by FimH in the absence of shear force results in a closing of the ligand-binding site, but, in contrast to selectins, is not directly linked to altered interdomain interactions. Here mechanical force promotes domain separation and completely releases FimH L from FimH P , which acts as an activator of ligand release via dynamic allostery. Remarkably, selectins and the fimbrial adhesin FimH thus employ entirely different mechanisms for establishing catch-bond behaviour by crosstalk between a lectin and an anchoring domain that provides tethering to a shaft. In both systems, the selectins and fimbrial adhesion, the shaft structures linking the terminal lectin/coupling domains to the cell surface, may contribute to the overall catch-bond behaviour, either via directly influencing coupling domain behaviour or via their general elastic properties [50] , [51] . The cell-tracking experiments indicate the importance of rapid ligand release from the high-mannose-type glycoprotein receptor uroplakin 1a in the lower urinary tract [52] for flagellar motility of piliated bacteria, and hence their ability to colonize new tissue areas under certain conditions during infection [12] , [29] , [53] . This provides a plausible explanation for the fact that low-affinity FimH variants were preserved in numerous uropathogenic E. coli strains. Binding of terminal mannoses with low affinity in the absence of shear force may also play a role in preventing the clearance of uropathogenic E. coli from the urinary tract by competitive binding to the Tamm–Horsfall protein in the urine [54] . In turn, populating the S bound state with an extremely low dissociation rate ensures tight bacterial adhesion under the mechanical forces of urine excretion. FimH is a promising target for anti-adhesive therapy of UTI because FimH antagonists, in contrast to antibiotics, are not exerting selection pressure towards resistance formation [18] , [55] , [56] . Previous ligand-binding studies on the isolated FimH L domain mimic the domain-separated S bound state of FimH. This state is characterized by extremely low off-rates and is promoted in vivo only after ligand-binding and the onset of flow conditions. Our kinetic data on ligand dissociation from full-length FimH demonstrate that rapid, competitive displacement of FimH from its carbohydrate ligands by FimH antagonists is well possible in the absence of shear force. Thus, full-length FimH (for example, in the form of the FimH·DsG complex established in this study) instead of the isolated FimH L domain is the relevant target for the development of anti-adhesive drugs. Importantly, the concept of the FimH·DsG model system can now be expanded to other related adhesive pilus adhesins. In combination with the novel fluorescent GN-FP-4 ligand, this model system paves the way for efficient screening for anti-adhesive drug candidates. Materials The synthetic DsG (sequence: ADVTITVNGKVVAKR) and DsF peptide (sequence: ADSTITIRGYVRDNG; >95% purity) were purchased from JPT (Germany). Guanidinium chloride (‘AA-Grade’ for spectroscopy) was obtained from NIGU Chemie (Germany). Standard chemical of highest purity available was obtained Sigma, Merck or AppliChem. If not mentioned otherwise, chromatography media for protein purification were purchased from GE Healthcare (UK). Oligonucleotides were from Microsynth (Switzerland). Construction of expression plasmids Expression plasmids for the periplasmic production of the E. coli F18 FimH lectin domain (FimH L F18 ) and for the periplasmic co-expression of full-length FimH F18 with FimC were based on the expression plasmids pfimH L and pfimH-fimC-ATG, respectively, for the analogous proteins from E. coli K12 (ref. 27 ). Six silent mutations replacing rare codons were introduced into the E. coli F18 fimH gene ( fimH F18 ) contained in the plasmid pGB2-24 (ref. 57 ) with the QuikChange mutagenesis kit (Agilent Technologies, Switzerland) to improve periplasmic expression. The coding sequence of the modified fimH F18 gene was amplified by PCR using the primers 5′-GATCCTCTAGAGGAGGGATGATTGTAATGAAACGAG-3′ and 5′-TTTCAAGCTTATTGATAAACAAAAGTCACG-3′ and cloned into pfimH-fimC-ATG [27] via the XbaI and HindIII sites (thereby replacing the fimH K12 gene) and yielded pfimH F18 –fimC–ATG. The gene encoding FimH L F18 was amplified with the primers 5′-GATCCTCTAGAGGAGGGATGATTGTAATGAAACGAG-3′ and 5′-CAGCCAAGCTTAGCCAGTAGGCACCACCAC-3′ and ligated via the XbaI and HindIII sites into ptrc99a-f1-stopp [27] . Protein production in the resulting plasmid pfimH L F18 is under control of the trc–promotor/ lac operator. Protein production and purification For purification of the complexes FimC·FimH K12 and FimC·FimH F18 , E. coli HM125 harbouring the corresponding co-expression plasmid was grown at 30 °C in 2YT medium containing ampicillin (100 μg ml −1 ). At an OD 600 of 1.5, isopropyl-β-D-thiogalactoside (IPTG) was added to a final concentration of 1 mM. The cells were further grown for 12−18 h, harvested by centrifugation, suspended in cold 50 mM Tris-HCl pH 7.5, 150 mM NaCl, 5 mM EDTA, 1 mg ml −1 polymyxin B sulfate (18 ml l −1 of culture) and stirred at 4 °C for 1.5 h. After centrifugation, the supernatant (periplasmic extract) was dialysed against 20 mM Tris-HCl pH 8.0 and applied to a QA52 (Whatman, Maidstone, UK) column equilibrated with the same buffer. The flow-through containing the respective FimC·FimH complex was dialysed against 20 mM MOPS–NaOH pH 7.0, loaded onto a Resource S column equilibrated with the same buffer and the complexes were eluted with a linear NaCl gradient (0−400 mM). Fractions containing FimC·FimH were pooled and loaded onto a Superdex 75 (HiLoad 26/60) column equilibrated with 20 mM NaH 2 PO 4 –NaOH pH 7.4, 50 mM NaCl. Fractions containing the pure complex were pooled and stored at 4 °C until further use. Typically, 3−5 mg of the purified complex were obtained per litre of bacterial culture. For expression of the isolated E. coli FimH L K12 and FimH L F18 , E. coli HM125 transformed with the respective expression plasmid was grown at 30 °C in M9 medium containing ampicillin (100 μg ml −1 ) to an OD 600 of 1.0, and expression was induced with 1 μM IPTG. After further growth for 12 h, cells were subjected to periplasmic extraction (see above). The extracts were mixed with 0.11 volumes of 1 M acetic acid–NaOH pH 4.5, dialysed against 10 mM acetic acid–NaOH pH 4.5 and then loaded onto a SP-Sepharose column equilibrated with the same buffer. The flow-through was collected and its pH was adjusted to 8.0 by addition of 1 M Tris-HCl pH 8.2. This solution was then applied to a Q-Sepharose column equilibrated with 20 mM Tris-HCl pH 8.0. The flow-through containing FimH L was loaded onto a Resource S column dialysed against 20 mM formic acid–NaOH pH 4.0. The protein was eluted with a linear NaCl gradient (0−1 M). Fractions containing pure FimH L were pooled, dialysed against water and stored at −20 °C. The identity of the purified proteins was confirmed by electrospray ionization (ESI)–mass spectrometry (FimH L F18 : calculated: 16,934.9 Da; measured: 16,935.0 Da; FimH L K12 : calculated: 16,963.0 Da; measured: 16,962.8 Da). About 11 mg of the pure FimH L was obtained per litre of bacterial culture. Production of FimH·DsG and FimH K12 ·DsF complexes The respective FimC·FimH complex (40 μM) was incubated with a threefold molar excess of the DsG peptide and incubated in 20 mM NaH 2 PO 4 –NaOH, pH 7.0, 50 mM NaCl for 48 h at 37 °C. The reaction mixture containing isolated FimC, the FimH·DsG complex and excess DsG was dialysed against 20 mM acetic acid–NaOH pH 4.5 and loaded onto a Resource S (6 ml) column equilibrated with the same buffer. The FimH·DsG complex was eluted with a linear NaCl gradient (0−400 mM). Fractions containing the pure complex were pooled, dialysed against water and stored at 4 °C. The FimH·DsG partially dissociated during ESI–mass spectrometry analysis, so that masses of the intact complexes and free FimH were obtained: FimH K12 ·DsG: calculated mass: 30,635.3 Da; measured mass: 30,636.0 Da; FimH F18 ·DsG: calculated mass: 30,607.3 Da; measured mass: 30,607.0 Da; FimH K12 : calculated mass: 29,064.5 Da; measured mass: 29,064.0 Da; FimH F18 : calculated mass: 29,036.4 Da; measured mass: 29,036.0 Da. The overall yields of the purified FimH·DsG complexes relative to the initial amount of FimC·FimH were in the range of 50–55%. The FimH K12 ·DsF complex was generated and purified as described for the FimH·DsG complexes (FimH K12 ·DsF: calculated mass: 30,702.2 Da; measured mass: 30,702.5 Da). The FimH·DsF complex was prepared from the FimC·FimH complex after mixing with DsF exactly according to the protocol described above for FimH·DsG and obtained in similar yields. Despite the non-natural interaction between FimH P and DsF, the FimH K12 ·DsF complex was formed four times faster than the FimH K12 ·DsG complex at pH 7.0 and 37 °C, with a rate constant of 2.2±0.5 M −1 s −1 . The FimH·DsF complex was stable against dissociation and unspecific aggregation. Determination of protein concentrations Protein concentrations were measured via the specific absorbance at 280 nm, using the following extinction coefficients (FimH K12 and FimH F18 have identical extinction coefficients): FimC·FimH (59,090 M −1 cm −1 ), FimH L (24,670 M −1 cm −1 ), FimH·DsG (35,090 M −1 cm −1 ) and FimH·DsF (36,580 M −1 cm −1 ). The concentrations of DsG and DsF were determined via their absorbance at 205 nm (42,650 and 49,700 M −1 cm −1 , respectively). Synthesis of the fluorescent-labelled FimH ligand GN-FP-4 To a stirred solution of mannoside 1 (25 mg, 0.061 mmol) [55] in dry dimethylformamide (DMF; 1 ml), N-hydroxysuccinimide (21 mg, 0.183 mmol) was added, followed by N,N′-dicyclohexylcarbodiimide (9.2 mg, 0.073 mmol). The mixture was stirred at room temperature for 2 h, then N -Boc-ethylendiamine (10.7 mg, 0.067 mmol) was added and the reaction was stirred for an additional 10 h. After cooling to 0 °C, the reaction mixture was diluted with water and concentrated. Chromatography on silica gel (CH 2 Cl 2 /MeOH) yielded 23 mg (0.042 mmol, 68%) of tert -butyl (3′-chloro-4′-(α-D-mannopyranosyloxy)-biphenyl-4-yl-carboxamido)ethyl)carbamate. This product was dissolved in CH 2 Cl 2 (3 ml) and trifluoroacetic acid (TFA, 1 ml) was added. The solid dissolved during addition of TFA. After 10 min at room temperature the reaction was complete. The mixture was evaporated and excess TFA was removed in high vacuum. The intermediate N -(2-aminoethyl)-3′-chloro-4′-(α-D-mannopyranosyloxy)-biphenyl-4-carboxamide TFA salt (23 mg, 0.042 mmol, quant.) was used without purification in the next step. After dissolution in dry DMF (0.5 ml), triethylamine (12.8 mg, 0.127 mmol) was added. The mixture was cooled to 0 °C, then fluorescein isocyanate (14.8 mg, 0.038 mmol) was added and the mixture was stirred for 3 h in the dark. After the addition of water, DMF was removed azeotropically, the residue dissolved in MeOH/10% acetic acid and evaporated. Chromatography on silica gel (CH 2 Cl 2 /MeOH) yielded compound 2 , contaminated with triethylammonium acetate. Therefore, after dissolution in MeOH, 0.5 N HCl in MeOH was added, the mixture evaporated and chromatographed on silica gel to yield pure compound GN-FP-4 ((3′-Chloro- N -(2-(3-(3′,6′-dihydroxy-3-oxo-3 H -spiro[isobenzofuran-1,9′-xanthen]-5-yl)-thioureido)ethyl)-4′-(α-D-mannopyranosyloxy)-biphenyl-4-carboxamide) [58] (15 mg, 47%). [α] D 20 +12.1 ( c 0.3, MeOH); 1 H NMR (500 MHz, CD 3 OD): δ =8.12 (s, 1H), 7.92 (d, J =8.3 Hz, 2H, Ar–H), 7.70 (dd, J =5.0, 13.1 Hz, 2H, Ar–H), 7.64 (d, J =8.3 Hz, 2H, Ar–H), 7.54 (dd, J =2.2, 8.6 Hz, 1H, Ar–H), 7.46 (d, J =8.7 Hz, 1H, Ar–H), 7.09 (d, J =8.2 Hz, 1H, Ar–H), 6.74 (s, 2H), 6.69 (d, J =1.4 Hz, 2H, Ar–H), 6.55 (d, J =8.4 Hz, 2H, Ar–H), 5.63 (d, J =1.3 Hz, H-1), 4.15 (dd, J =1.8, 3.1 Hz, H-2), 4.03 (dd, J =3.4, 9.5 Hz, H-3), 3.94 (s, 2H, CH 2 ), 3.86-3.64 (m, 6H, H-4, H-5, H-6, CH 2 ); 13 C NMR (126 MHz, CD 3 OD): δ =153.21, 143.84, 136.41, 129.66, 129.18, 127.76, 127.70, 125.37, 118.64, 103.62 (Ar-C), 100.75 (C-1), 76.00 (C-5), 72.41 (C-3), 71.86 (C-2), 68.24 (C-4), 62.69 (C-6), 40.76 (CH 2 ); ESI–MS: m/z : Calculated for C 42 H 37 ClN 3 O 12 S [M+H] + : 842.2, found: 842.2. Fluorescence spectroscopy Fluorescence emission spectra of FimH variants were recorded between 300 and 450 nm (excitation at 280 nm) at 25 °C in 1.0 × 0.4-cm quartz cuvettes on a QM 7/2003 spectrofluorimeter (PTI, USA) equipped with a magnetic stirrer. Protein concentrations were 1−2 μM in 20 mM MOPS–NaOH pH 7.4. Fluorescence spectra of GN-FP-4 ( ɛ 495 nm =54,900 M −1 cm −1 ) were recorded between 500 and 650 nm (excitation at 497 nm) in the same buffer. Kinetics of HM binding to FimH·DsG The rate constants of binding ( k on ) and dissociation ( k off ) for the complex between FimH·DsG and HM were measured at 25 °C in 20 mM MOPS–NaOH pH 7.4 in a SX20 stopped-flow instrument (Applied Photophysics, UK). A constant FimH·DsG concentration of 1 or 2 μM was used. FimH·DsG was mixed with different concentrations of HM (2−100 μM), and binding was monitored by the increase in fluorescence above 320 nm (excitation at 280 nm). The fluorescence traces were globally fitted with Dynafit [59] according to a second-order binding and first-order dissociation reaction. As an additional control, the fluorescence amplitudes of the individual reactions were plotted against the total HM concentration and fitted according to equation (2). The deduced dissociation constants reproduced the K d values obtained with equilibrium titration within experimental error. Equilibrium titration of FimH·DsG with HM The binding equilibrium between FimH·DsG and HM was followed at 25 °C in 20 mM MOPS–NaOH pH 7.4 on a QM 7/2003 spectrofluorometer (PTI) by the increase in fluorescence at 320 nm on HM binding (excitation at 280 nm). Measurements were performed with a stirred 1 × 0.4-cm quartz cuvette. The concentration of FimH·DsG was kept constant at 2 μM and the concentration of HM was varied between 0 and 200 μM. The samples were equilibrated overnight, and their fluorescence intensities were recorded for 30 s and averaged. The fluorescence intensities were plotted against total HM concentration and fitted according to equation (2) where F is the monitored fluorescence signal, F 0 is the fluorescence signal in absence of ligand, F ∞ is the fluorescence signal at full saturation with ligand, K d is the dissociation constant, [P] 0 is the total concentration of FimH·DsG and [L] 0 is the total concentration of HM. Equilibrium titration of FimH L with GN-FP-4 The binding equilibrium between FimH L and GN-FP-4 at 25 °C in 20 mM MOPS–NaOH pH 7.4, supplemented with 0.001% Tween 20 to prevent unspecific adsorption effects at nanomolar concentrations, was recorded by the decrease in GN-FP-4 fluorescence at 520 nm (excitation at 497 nm). Measurements were performed with a stirred 1 × 0.4-cm quartz cuvette. The concentration of GN-FP-4 was kept constant at 1.0 or 2.0 nM and the concentration of FimH L was varied between 0 and 10 nM. The samples were equilibrated overnight, and their fluorescence intensities at 520 nm were recorded for 30 s and averaged. The experimental data were fitted according to equation (2). Displacement of HM from the FimH L by GN-FP-4 The rate constant of dissociation ( k off ) for HM from FimH L at 25 °C in 20 mM MOPS–NaOH pH 7.4 was measured indirectly by binding of excess GN-FP-4 to FimH L after dissociation of HM, recorded with the decrease in GN-FP-4 fluorescence at 520 nm (excitation at 497 nm). A mixture of FimH L and HM (3 μM each), pre-incubated for at least 18 h, was mixed with different amounts of excess GN-FP-4 (final concentrations: 10−40 μM), and GN-FP-4 fluorescence was recorded every 10 min for 10 s, averaged and the data fitted according to first-order kinetics. The obtained rate constants were independent of GN-FP-4 concentration and thus identical to the dissociation rate of HM from FimH L . Determination of the FimH L ·HM dissociation constant The affinity of FimH L for HM at 25 °C in 20 mM MOPS–NaOH pH 7.4 was determined by the competition between HM and GN-FP-4 for binding to FimH L . A mixture of FimH L and GN-FP-4 (1 μM each) was incubated with different concentrations of HM (10–3.2 mM) and incubated for at least 18 h. The displacement of GN-FP-4 by HM was recorded on by the decrease in the fluorescence polarization at 528±20 nm (excitation at 485±20 nm) on a microplate reader (Biotek, USA), using flat black-bottom 96-well microtitre plates (Greiner, Austria). The fluorescence polarization data were fitted with Dynafit [59] according to an equilibrium competition mechanism, with the total concentrations of FimH L , GN-FP-4 and HM (variable) and the respective K d of GN-FP-4 ( Table 2 ) as input, and K d of HM and the fluorescence polarization at zero and infinite HM concentration as open parameters. Crystallization of FimH variants All crystallization experiments were performed at 4 °C with the sitting drop vapour diffusion method. For crystallization, FimH F18 ·DsG and FimH K12 ·DsG (0.1−0.2 μl, 15 mg ml −1 in H 2 O) was mixed with 0.1−0.2 μl of precipitant (25% (w/v) polyethylene glycol (PEG) 3350, 0.2 M magnesium chloride, 0.1 M BisTris-HCl pH 5.5 at 4 °C. Crystals of FimH F18 ·DsG and FimH K12 ·DsG grew within 4−6 weeks and are of the space group C2, with one molecule per asymmetric unit. FimH K12 ·DsG crystals in space group P1 grew at 0.2 M Na Malonate, 20% PEG3350 within 2 months at 4 °C. For crystallization of the FimH F18 ·DsG·HM complex, a threefold excess over FimH·DsG was used (protein concentration and protein/precipitant ratios were as described for FimH·DsG). Crystals of the space group P2 1 3 appeared after 1 month in 30% (v/v) 2-Methyl-2,4-pentanediol, 0.1 M sodium cacodylate, 0.2 M magnesium acetate pH 6.5 at 4 °C. FimH K12 ·DsF·HM crystals appeared after 2 months in 30% w/v PEG 5000, 0.1 M 2-( N -morpholino)ethanesulfonic acid (MES) monohydrate, 0.2 M ammonium sulfate pH 6.5 at 20 °C (2.5-fold excess of ligand over protein). FimH L F18 ·HM crystallized in 17% PEG 2000 MME, 0.1 M HEPES–NaOH pH 7.5 at 4 °C. FimH L K12 ·HM crystallized in 1.5 M (NH4) 2 SO 4 , 0.2 M Na acetate pH 5.5 at 20 °C. Crystallographic data collection All crystals, except for FimH F18 ·DsG·HM, were cryo-preserved by the addition of ethane-1,2-diol to a final concentration of 20% (v/v). The precipitant solution used for the crystallization of FimH F18 ·DsG·HM already contained 30% (v/v) methyl-2,4-pentanediol, which acts as cryoprotectant. Crystals were flash-cooled in liquid nitrogen. All measurements were carried out at the SLS beamline X06DA and X06SA (Swiss Light Source, Paul Scherrer Institute, Switzerland) at 100 K. All data were integrated, indexed and scaled using the XDS software package [60] (5% of the reflections were set aside as test set). Data collection statistics are summarized in Table 1 . Crystallographic structure determination All structures were solved by molecular replacement using structures of isolated FimH L (AA1-158, PDB ID: 3MCY [18] , and the pilin domain of FimC·FimH (AA160-297, PDB ID: 1QUN [24] , as search models with the programme Phaser [61] ). Model building and structure refinement were performed with Coot (ref. 62 ) and PHENIX (ref. 63 ). Twelve out of thirteen residues could be built for the FimG donor strands in the crystal structures, and only the C-terminal lysine residue had weak electron density. Refinement statistics are summarized in Table 1 . Molecular dynamics simulations Four molecular systems were prepared for FimH F18 . The first system was constructed using the A bound state of FimH F18 ·DsG·HM ( Supplementary Fig. 3a,b ) and the second system is equivalent but HM was removed ( Supplementary Fig. 3c,d ). The third system contains only the FimH L and HM from the A bound X-ray structure ( Supplementary Fig. 3e,f ). The fourth system was prepared for FimH L and HM based on the S bound state in the FimH K12 ·DsF·HM crystal structure ( Supplementary Fig. 3g,h ). The CHARMM-GUI web server [64] was used to prepare the molecular systems, which were solvated with TIP3 water molecules and ionized with 50 mM NaCl. Each system contains between 50,000 and 60,000 atoms. All simulations were performed with the NAMD simulation package (version 2.9) (ref. 65 ). The CHARMM36 force field was used for the protein, and parameters for HM were generated using the CHARMM General Force Field programme (version 0.9.7 beta). Electrostatic interactions were calculated using the particle-mesh Ewald method [66] with a grid spacing of 1 Å. The cutoff for the van der Waals interactions was taken at 12 Å with a switching function used after 10 Å. Time step for the integration of dynamics was 2 fs. Simulations were performed in an isothermal–isobaric ensemble, with a pressure of 1 atm and a temperature of 300 K. Cell tracking on mannose–BSA-coated surfaces The E. coli KB18 strain [67] was kindly provided by Professor Evgeni Sokurenko and served as host for the generation of recombinant strains. KB18 contains the pPKL114 plasmid [57] , which encodes the whole fim operon with a translational stop linker upstream of the fimH gene. KB18 was co-transformed with the pGB2-24 plasmid, which was isolated from the ELT115 strain and encodes fimH J96 (kindly provided by Professor Evgeni Sokurenko). Single-nucleotide point mutations were introduced in fimH J96 using overlap extension PCR following standard molecular techniques to obtain fimH F18 and fimH F18 -Ala188Asp. The PCR products were cloned into pGB2-24 by the ApaLI and SphI sites, and KB18 was transformed with the resulting plasmid. E. coli strains were grown from frozen stocks in LB medium supplemented with antibiotics (100 μg ml −1 ampicillin and 25 μg ml −1 chloramphenicol) until late log phase (OD 600 of 1.0–1.2) and diluted to an OD 600 of 0.01 before movie acquisition. Cell culture dishes (35 mm, Corning Inc., Corning, NY) were incubated with 50 μl of 50 μg ml − 1 1M-BSA in 0.02 M bicarbonate buffer for 75 min at 37 °C. The dishes were then washed three times and quenched with 0.1% PBS–BSA to remove unbound 1M-BSA and block remaining sites on the plastic surface to prevent nonspecific binding of bacteria. Controls were prepared by treating cell culture dishes with 0.1% PBS–BSA only. The bacterial suspension was added to the cell culture dishes for microscopy studies. Cell tracking was carried out at room temperature under static conditions. A bacterial suspension of 50 μl in the late logarithmic growth phase was placed onto the cell culture dishes (diluted to OD 600 of 0.01), and a cover slide was placed on top. The delay between sample placement and start of the movie acquisition was about 1 min. Time-lapse movies were recorded with a × 20 phase contrast objective using a CMOS digital camera (The Imaging Source Europe, Bremen, Germany) mounted on a Nikon Ti Eclipse inverted microscope and using the NIS Elements Basic Research software (Nikon, Zurich, Switzerland). Phase contrast images in an ∼ 5-μm-thick surface layer were taken at four to five frames per second over 5 min. The dead time of movie acquisition was ∼ 1 min. The resulting images were segmented by creating a projection of the average intensities over all frames to remove the background and by subsequent thresholding using the Maximum Entropy method in Fiji [68] to obtain binary images (examples shown in Supplementary Movies 1 and 2 ). The segmented movies were imported into Imaris (Bitplane, Zurich, Switzerland) and tracked through the autoregressive algorithm. A time filter was applied to exclude all tracks with a length below 15 s. Tracks longer than 15 s were reviewed individually and edited manually, if necessary. Five to seven independent movies were recorded for each experimental set-up: FimH F18 or FimH F18 -Ala188Asp on 1M-BSA-coated dishes and FimH F18 and FimH F18 -Ala188Asp on BSA-coated cell culture dishes. E. coli piliated with FimH F18 or FimH F18 -Ala188Asp binding to 1M-BSA in the absence (1,815 and 1,283 individual tracks, respectively) and in the presence of 200 μM HM (1,175 and 1,071 individual tracks, respectively) were analysed respectively. For E. coli piliated with FimH F18 or FimH F18 -Ala188Asp binding to BSA 1,314 and 1,065 individual tracks, respectively, were analysed. Bacteria with a speed of <0.5 μm s −1 were classified as attached, all other bacteria were classified as mobile. Owing to limitation in the spatial and temporal resolution of movie acquisition, we did not further subdivide bacterial swimming into motility behaviours as ‘rolling’ [29] , [53] , ‘roaming’, ‘orbiting’ and so on. The individual cell tracks were classified into four classes: no motility change during observation (pre-attached or mobile), transient attachment, permanent attachment and permanent detachment. For FimH F18 on 1M-BSA surfaces, 13.9% (251 out of 1,815 tracks) of all tracks showed a single transient attachment event ( Supplementary Fig. 7d ). In total, 67 out of the 251 bacteria that underwent a first transient adhesion attached and detached from the surface a second time. For these cells, the average time between detachment and re-attachment was only 13.5 s ( Supplementary Fig. 7e ), suggesting that re-binding may be favoured by proximity to the surface as compared with the initial attachment. The mean velocity on 1M-BSA, as compared with BSA-coated surfaces, was reduced for both FimH F18 -piliated (4.2 and 7.4 μm s −1 , respectively) and FimH F18 –Ala188Asp-piliated bacteria (3.5 and 8.1 μm s −1 , respectively; Supplementary Fig. 7a,b ). This reduction of the mean velocity originates from two different phenomena: in FimH F18 -piliated cells it is caused by a change from fast swimming to a slower mode of motion ( Supplementary Fig. 7b ; Supplementary Movie 1 ), which is consistent with bacterial surface rolling due to weak, short-lived mannose-based interactions [29] , [53] . In contrast, for FimH F18 –Ala188Asp-piliated bacteria, the reduction of the mean velocity results from an increase in the fraction of adherent cells on 1M-BSA compared with BSA (see main text). In the presence of 200 μM HM, the mean velocity on 1M-BSA is increased for both FimH F18 -piliated (6.5 μm s −1 ) and FimH F18 –Ala188Asp-piliated bacteria (5.9 μm s −1 ; Supplementary Fig. 7a ) and transient and permanent attachment is reduced by 75% and 85%, respectively ( Fig. 6 and Supplementary Fig. 7c ). Accession codes: The atomic coordinates and structure factors have been deposited in the Protein Data Bank under the accession codes 4XO8, 4XO9, 4XOA, 4XOB, 4XOC, 4XOD, 4XOE. How to cite this article: Sauer, M. M. et al. Catch-bond mechanism of the bacterial adhesin FimH. Nat. Commun. 7:10738 doi: 10.1038/ncomms10738 (2016).